Aharonov–Bohm oscillations in a quasi-ballistic three-dimensional topological insulator nanowire Aharonov–Bohm oscillations effectively demonstrate coherent, ballistic transport in mesoscopic rings and tubes. In three-dimensional topological insulator nanowires, they can be used to not only characterize surface states but also to test predictions of unique topological behaviour. Here we report measurements of Aharonov–Bohm oscillations in (Bi 1.33 Sb 0.67 )Se 3 that demonstrate salient features of topological nanowires. By fabricating quasi-ballistic three-dimensional topological insulator nanowire devices that are gate-tunable through the Dirac point, we are able to observe alternations of conductance maxima and minima with gate voltage. Near the Dirac point, we observe conductance minima for zero magnetic flux through the nanowire and corresponding maxima (having magnitudes of almost a conductance quantum) at magnetic flux equal to half a flux quantum; this is consistent with the presence of a low-energy topological mode. The observation of this mode is a necessary step towards utilizing topological properties at the nanoscale in post-CMOS applications. In three-dimensional topological insulator (3D TI) nanowires, charge transport occurs via gapless surface states where the spin is fixed perpendicular to the momentum [1] , [2] , [3] , [4] , [5] , [6] . When a magnetic field ( B ) is applied along the nanowire axis, the surface electrons encircling the wire pick up a phase of 2 π Φ/Φ 0 , where Φ= BS is the magnetic flux through cross-sectional area S and Φ 0 = h/e is the magnetic flux quantum, where h is Planck’s constant and e the electron charge. The energy–momentum relation is, thus, periodic in Φ/Φ 0 , leading to h / e Aharonov–Bohm (AB) oscillations [7] , [8] , [9] . In topological insulators, the spin-momentum locking causes carriers encircling the wire to also acquire a π Berry phase, which is predicted to open up a gap in the lowest-energy one-dimensional (1D) surface sub-band. Inserting a magnetic flux of h /2 e through the nanowire should cancel the Berry phase and restore the gapless 1D mode [10] , [11] . Thus, the topological nature of the 1D surface sub-bands can be observed via the behaviour of the AB oscillation maxima and minima as a function of Φ/Φ 0 : for the lowest-energy mode (at the Dirac point), a minimum in conductance should occur at Φ/Φ 0 =0, while a maximum in conductance should occur at Φ/Φ 0 =0.5, as the non-degenerate gapless mode reappears [10] , [11] . This mode contains massless Dirac-like excitations that follow a 1D linear energy–momentum dispersion, and is not observed in non-topological systems [7] , [8] , [9] , [12] . Previous experiments have demonstrated AB oscillations in 3D TI nanowires, indicating surface transport [13] , [14] , [15] . However, the predicted behaviour close to the Dirac point has not been observed. The experiments performed here differ in several significant ways. First, excess n -doping was removed using the chemical dopant 2,3,5,6-tetrafluoro-7,7,8,8-tetracyanoquinodimethane, allowing transport to be measured, while E F is tuned through the Dirac point [1] , [16] . Second, the small sample sizes used here allow for quasi-ballistic transport. In the quasi-ballistic regime, h / e AB oscillations are predicted to dominate over h /2 e Aharonov–Altshuler–Spivak (AAS) oscillations [9] , [10] , [12] . AAS oscillations originate from interference between time-reversed paths due to weak (anti)localization and, thus, differ from AB oscillations in their physical origin. In the quasi-ballistic regime, the channel length ( L ) should not be much longer than the mean-free path ( l m ). In addition, L should be long enough for the electrons to circumnavigate the nanowire before exiting the channel, to observe dependence of the conductance on a magnetic flux. Here we report measurements of low-doped, quasi-ballistic, mechanically exfoliated 3D TI nanowires. The use of these devices allows us to observe alternations of conductance maxima and minima with carrier density; in particular, we observe a minimum conductance at Φ=0 and a maximum conductance close to e 2 / h at Φ= h /2 e near the lowest sub-band (that is, the Dirac point). This behaviour is consistent with topological surface transport, and thus marks a step towards utilizing topological properties at the nanoscale in applications such as quantum computing and information processing architectures. Quasi-ballistic devices near the Dirac point Our samples are exfoliated from a TI crystal (Bi 1.33 Sb 0.67 )Se 3 . Angle-resolved photoemission spectroscopy of the crystal shows a bulk conduction band located ∼ 0.20 eV above the Dirac point, as well as gapless linear surface states inside the bulk bandgap [16] . Previous results on similar samples [16] demonstrate that the resistance maximum coincides well with the charge neutrality point, and that the discrepancy, in gate voltage, between these and the Dirac point should be less than 1V. Nanowires are obtained via mechanical exfoliation of a bulk TI crystal (Bi 1.33 Sb 0.67 )Se 3 onto Si/SiO 2 substrates, where the doped substrate acts as a global backgate (see Methods). While chemical or mechanical etching allows for effective production of nanowires from layered thin films, these processes typically introduce additional damage and defects along the edges [17] , [18] . We fabricated two four-terminal devices having channel lengths of L 1 =200 nm and L 2 =350 nm (see Fig. 1a,b ). The 200-nm device has width=110 nm and thickness=15 nm ( S 1 =1.65 × 10 −15 m 2 ), while the 350 nm device has width=100 nm and thickness=16 nm ( S 2 =1.60 × 10 −15 m 2 ). The typical mean-free path l m ≈100 nm of the nanowires is estimated from the gate-dependent conductivity of the surface electrons using l m = v F τ and , where v F is the Fermi velocity, σ the conductivity, n the carrier density, ħ is the reduced Planck’s constant and e is the electron charge. Thus, both devices are in the quasi-ballistic regime where L / l m ∼ 2–3 (ref. 19 ). Samples were measured using standard four-terminal lock-in techniques in a dilution refrigerator at the base temperature of 16 mK. 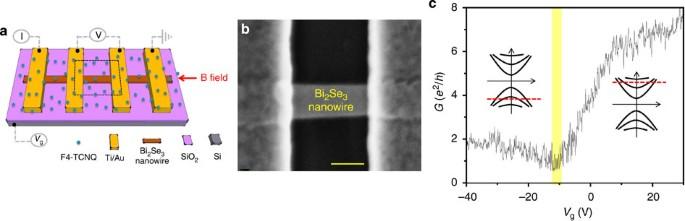Figure 1: Device configuration and characterization. (a) Device and measurement schematic showing four-point lead configuration and chemical dopant, F4-TCNQ. (b) Scanning electron microscope image of the 200-nm device, corresponding to dashed region ofa. Scale bar, 100 nm. (c) Four-terminal conductanceGas a function of back-gate voltageVgatB=0 andT=16 mK. The conductance minimum indicates the location of the Dirac point atVg≈−12 V (yellow-shaded region: −13 V<Vg<−11 V). Inset schematics indicate the position ofEFin either the conduction or valence band. F4-TCNQ, 2,3,5,6-tetrafluoro-7,7,8,8-tetracyanoquinodimethane. Figure 1c shows the location of the Dirac point for the 200-nm device at V g ≈−12 V, and demonstrates that the Fermi energy can be tuned through the Dirac point with a back-gate voltage. It has been shown that when the initial doping level is low in nanostructured TI devices, the Fermi energies of the top and bottom surfaces can be simultaneously tuned with a single gate electrode, due to the large inter-surface capacitance [1] ; as will be discussed below, even if a slight chemical potential mismatch between the top and bottom surface states does occur, it does not significantly affect the AB behaviour. The fluctuations evident in Fig. 1c are reproducible universal conductance fluctuations, which can affect the magnitude of conductance at fixed gate voltage; however, the conductance minimum ∼ −12 V is still apparent. Figure 1: Device configuration and characterization. ( a ) Device and measurement schematic showing four-point lead configuration and chemical dopant, F4-TCNQ. ( b ) Scanning electron microscope image of the 200-nm device, corresponding to dashed region of a . Scale bar, 100 nm. ( c ) Four-terminal conductance G as a function of back-gate voltage V g at B =0 and T =16 mK. The conductance minimum indicates the location of the Dirac point at V g ≈−12 V (yellow-shaded region: −13 V< V g <−11 V). Inset schematics indicate the position of E F in either the conduction or valence band. F4-TCNQ, 2,3,5,6-tetrafluoro-7,7,8,8-tetracyanoquinodimethane. Full size image Aharonov-Bohm oscillations as a function of Fermi energy The band structure of surface carriers in a 3D TI nanowire is described by a 1D momentum vector k along the nanowire axis. The 1D sub-bands in the presence of an axial magnetic field are described by [14] , [20] : Here, is a (half integer) angular momentum, v F is the Fermi velocity, and S is the cross-sectional area of the nanowire. 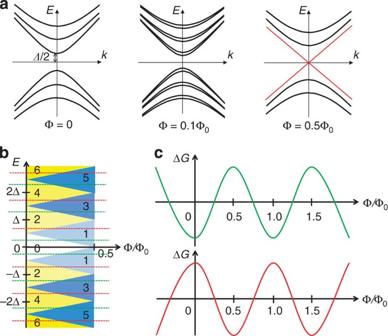Figure 2: Schematics of TI nanowire band structure and magnetoconductance. (a) Schematic band structure of a TI (Bi2Se3) nanowire at Φ/Φ0=0, 0.1 and 0.5, showing the appearance of the low-energy topological mode at Φ/Φ0=0.5. The sub-band spacing, Δ, for Φ=0 andk=0 is labelled. (b) 1D sub-band occupancy for varying chemical potential,EF, as a function of Φ/Φ0. The coloured regions and related numbers show the occupancy of sub-band modes, which increases with Δ, and can change with Φ as the sub-band spacing varies with respect toEF. (c) Expected alternating patterns of magnetoconductance (ΔG) oscillations withEF. Green and red lines curves correspond to same colour dashed lines inb. Figure 2a depicts schematic band structures for Φ/Φ 0 =0, 0.1 and 0.5. The 1D sub-bands are gapped at Φ/Φ 0 =0 by Δ, where . While all the sub-bands at Φ/Φ 0 =0 are doubly degenerate, the degeneracy becomes lifted at Φ/Φ 0 ≠0. The behaviour of the AB oscillations should also vary with carrier density [21] , which can be tuned by an external voltage. In Fig. 2b , a schematic mapping shows the number of modes at various Fermi energies, E F . At | E F |<Δ/2, the number of modes at Φ/Φ 0 =0 and 0.5 should be 0 and 1, respectively. Therefore, in a ballistic transport regime, the conductance should exhibit a minimum at Φ/Φ 0 =0 and a maximum of ≈ e 2 / h at Φ/Φ 0 =0.5. Away from the Dirac point the phase of the conductance alternates: when E F is located at one of the green(red)-dotted lines in Fig. 2b , the conductance should have a minimum(maximum) at Φ/Φ 0 =0 and a maximum(minimum) at Φ/Φ 0 =0.5, as depicted in Fig. 2c . Figure 2: Schematics of TI nanowire band structure and magnetoconductance. ( a ) Schematic band structure of a TI (Bi 2 Se 3 ) nanowire at Φ/Φ 0 =0, 0.1 and 0.5, showing the appearance of the low-energy topological mode at Φ/Φ 0 =0.5. The sub-band spacing, Δ, for Φ=0 and k =0 is labelled. ( b ) 1D sub-band occupancy for varying chemical potential, E F , as a function of Φ/Φ 0 . The coloured regions and related numbers show the occupancy of sub-band modes, which increases with Δ, and can change with Φ as the sub-band spacing varies with respect to E F . ( c ) Expected alternating patterns of magnetoconductance (Δ G ) oscillations with E F . Green and red lines curves correspond to same colour dashed lines in b . Full size image The magnetoconductance at the Dirac point of the 200-nm device is plotted as a function of Φ/Φ 0 in Fig. 3a . The magnetoconductance clearly shows h / e AB oscillations, for flux through an area consistent with the measured cross-section of the nanowire. The fast Fourier transform of the data ( Fig. 3b ) confirms the predominant h / e AB and absent h /2 e AAS oscillations, implying quasi-ballistic, phase-coherent transport along the device. Quasi-ballistic behaviour is further confirmed by the observation of Fabry–Perot oscillations [22] , [23] , [24] , [25] in similar TI nanowire devices (see Supplementary Fig. 1 and Supplementary Note 1 ). We observe maximum conductance values close to e 2 / h (≈0.9 e 2 / h ) at Φ/Φ 0 =0.5. Moreover, the magnetoconductance minimum near Φ/Φ 0 =0 and maximum near Φ/Φ 0 =0.5 are consistent with the presence of a low-energy topological mode [10] , [11] , [22] . Similar magnetoconductance minimum at Φ/Φ 0 =0 and maximum≈ e 2 / h at Φ/Φ 0 =0.5 were observed in the 350-nm device, as well as for the 200-nm device in different thermal cycles (see Supplementary Figs 2 and 3 , and Supplementary Note 2 ). This reproducibility suggests that the behaviour of the AB oscillations at the Dirac point is a robust phenomenon. 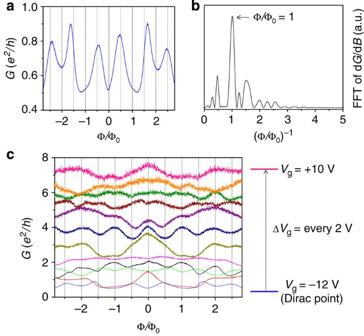Figure 3: Magnetoconductance data for 200-nm device. (a) Magnetoconductance measured at the Dirac point (Vg≈−12 V), showing AB oscillations with a period of Φ/Φ0=1. A conductance minimum occurs at Φ/Φ0=0. (b) Fast Fourier transform of dG/d(Φ/Φ0) fromashowing dominant AB (h/e) and lack of AAS (h/2e) oscillations. (c) Magnetoconductance measured away from the Dirac point showing alternating phase of AB with gate voltageVg. ConductanceGversus magnetic flux Φ/Φ0is measured fromVg=−12 V (Dirac point) to +10 V, in steps of 2 V. Note that no background has been removed from this data. Figure 3: Magnetoconductance data for 200-nm device. ( a ) Magnetoconductance measured at the Dirac point ( V g ≈−12 V), showing AB oscillations with a period of Φ/Φ 0 =1. A conductance minimum occurs at Φ/Φ 0 =0. ( b ) Fast Fourier transform of d G /d(Φ/Φ 0 ) from a showing dominant AB ( h / e ) and lack of AAS ( h /2 e ) oscillations. ( c ) Magnetoconductance measured away from the Dirac point showing alternating phase of AB with gate voltage V g . Conductance G versus magnetic flux Φ/Φ 0 is measured from V g =−12 V (Dirac point) to +10 V, in steps of 2 V. Note that no background has been removed from this data. Full size image Figure 3c shows the magnetoconductance for increasing gate voltages, demonstrating that the AB phase alternates with an approximate period of Δ V g =2 V. This is consistent with the phase alternations predicted to occur periodically when E F increases by half the sub-band spacing, or ½ Δ (refs 10 , 11 ). Similar phase alternations with gate voltage were observed in the 350-nm device (see Supplementary Figs 2 and 3 and Supplementary Note 2 ). Due to the limited resolution in gate voltage steps (limited by voltage jumps due to local charging effects), Fig. 3c may not show all the alternating phases of the AB oscillations; however, the overall dependence of the magnetoconductance on gate voltage is qualitatively consistent with theoretical expectations [10] , [11] . Because sub-bands away from the Dirac point may be diffusive, the amplitudes of AB oscillations in these regions vary between 0 and e 2 / h (refs 11 , 19 ). At the Dirac point, a perfectly transmitted mode is predicted to contribute e 2 /h to the conductance [10] , [11] when Φ/Φ 0 =0.5. We observe a conductance maximum near the Dirac point of ≈0.9 e 2 / h at Φ/Φ 0 =0.5. The reason for this discrepancy is unclear. It is possibly caused by variations due to universal conductance fluctuations in the nanowire, or the effects of macroscopic irreversibility brought about by quasiparticles that enter and are emitted from the metallic voltage probes [19] , [26] . The data also show finite conductance (≈0.5 e 2 / h in Fig. 3a ) at Φ/Φ 0 =0 in the gapped nanowire near the Dirac point. This could occur if chemical potential fluctuations due to strong disorder were much larger than the gap size [10] , [11] . However, in that case, h /2 e AAS oscillations would dominate over h / e AB oscillations, which is inconsistent with our observations. Rather, the finite conductance at Φ/Φ 0 =0 is likely due to small deviations of E F from the Dirac point, as discussed below. The data further show that the phase of the AB oscillations becomes less regular at large magnetic field, which is likely due to the Zeeman energy. At low magnetic field, the Zeeman energy is negligible compared with the energy spacing of sub-bands: in the 200-nm device at Φ/Φ 0 =0.5, where g ≈23 is the g-factor. However, at large B (Φ/Φ 0 >2) the Zeeman energy is comparable to Δ. The magnetoconductance data can be better understood by comparing it with full 3D simulations of TI nanowires coupled with the metallic contacts, calculated within the non-equilibrium Green’s function formalism [19] (see Supplementary Note 3 ). 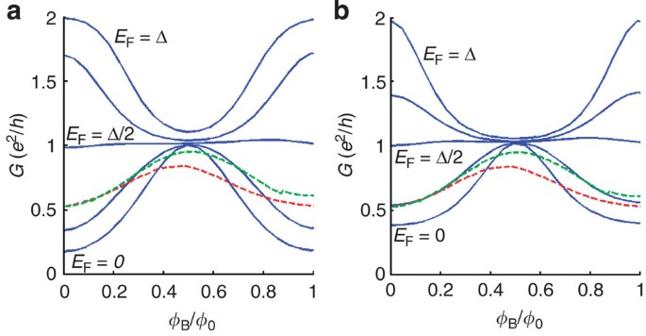Figure 4: Simulated magnetoconductance. (a) AB oscillations for a TI nanowire forEFranging from the Dirac point to Δ in increments of Δ/4. The conductance atG(Φ/Φ0=0) increases with increasingEF. The Dirac point conductanceG(Φ/Φ0=0)=0.20e2/hemerges due to evanescing modes from the metallic contacts, although this effect is enhanced in the simulations due to the short channel length. Experimental magnetoconductance from the 200-nm device (red-dashed curve) and the 350-nm device (green-dashed curve) are overlaid. (b) AB oscillations for a TI nanowire with a linear band bending profile of 2Δ for the sameEFvalues asashowing a further increase in conductance atG(Φ/Φ0=0). The simulations show good qualitative agreement with the overlaid experimental data. Figure 4 plots simulated magnetoconductance for a series of E F ranging from the Dirac point to Δ, demonstrating the AB phase alternation with increasing E F . Figure 4a shows finite zero-field conductance due to off-resonant transmission, which can occur when short wires are coupled with metallic contacts. The simulations indicate that increasing E F only a few meV from the Dirac point can add a significant fraction of e 2 /h to zero-field conductance. For example, G (Φ/Φ 0 =0) increases from 0.20 e 2 / h to 0.45 e 2 / h when E F shifts from the Dirac point to Δ/4 (a shift of ≈3.6 meV for the 200-nm device). In addition, zero-field conductance can be lifted by any band bending brought about by the chemical dopant, which can effectively add a linear chemical potential across the thickness of the nanowire. Although the chemical doping method we employ is not expected to produce significant band bending in Bi 2 Se 3 (ref. 1 ), the nanowire magnetoconductance is very sensitive to slight deviations in chemical potential, due to the small surface state band gap. For example, Fig. 4b shows that band bending of 30 meV≈2Δ can yield finite conductance at Φ/Φ 0 =0, at both the Dirac point and Δ/4. Although it is difficult to distinguish the relative experimental magnitude of each contribution, Fig. 4b shows that a combination of these two effects can fully account for the zero-field conductance near the Dirac point, and leads to a good qualitative agreement between theory and experiment. Figure 4: Simulated magnetoconductance. ( a ) AB oscillations for a TI nanowire for E F ranging from the Dirac point to Δ in increments of Δ/4. The conductance at G (Φ/Φ 0 =0) increases with increasing E F . The Dirac point conductance G (Φ/Φ 0 =0)=0.20 e 2 /h emerges due to evanescing modes from the metallic contacts, although this effect is enhanced in the simulations due to the short channel length. Experimental magnetoconductance from the 200-nm device (red-dashed curve) and the 350-nm device (green-dashed curve) are overlaid. ( b ) AB oscillations for a TI nanowire with a linear band bending profile of 2Δ for the same E F values as a showing a further increase in conductance at G (Φ/Φ 0 =0). The simulations show good qualitative agreement with the overlaid experimental data. Full size image By fabricating quasi-ballistic 3D TI nanowire devices that are gate tunable through the Dirac point, we have been able to demonstrate salient features of AB oscillations not seen in other non-topological nanowire systems. In particular, we observe alternations of conductance maxima and minima with gate voltage, and, at the Dirac point, conductance minima near Φ/Φ 0 =0 with corresponding maxima of ∼ e 2 / h near Φ/Φ 0 =0.5, which is consistent with the existence of a low-energy topological mode. The observation of this mode is a necessary step towards utilizing topological properties at the nanoscale in post-complementary metal-oxide-semiconductor (CMOS) applications, for example, in topological quantum computing devices [27] or as efficient replacements for metallic interconnects in information processing architectures [28] . Device fabrication and measurement Three-dimensional TI crystals (Bi 1.33 Sb 0.67 Se 3 ) were grown using a modified floating zone method [16] . TI nanowires were obtained by mechanical exfoliation (‘scotch tape method’) of bulk (Bi 1.33 Sb 0.67 )Se 3 crystals on 300 nm SiO 2 /highly n -doped Si substrates [29] . The nanowires were identified via optical and atomic force microscopy [1] , [30] , [31] . Nanowire thickness was determined by atomic force microscopy, while the width was more accurately determined by scanning probe microscopy after all electrical measurements were completed. After the nanowires were located on the SiO 2 /Si chips, electron beam lithography was performed to define four-point electrodes. Subsequently, the surface was cleaned with brief ion milling and Ti(2.5 nm)/Au(50 nm) were deposited at a base pressure ≈1 × 10 −9 torr. Immediately after lift-off, ∼ 14 nm of 2,3,5,6-tetrafluoro-7,7,8,8-tetracyanoquinodimethane (Sigma-Aldrich) was deposited via thermal evaporation. Finally, the devices were wire bonded and cooled down in a commercial dilution refrigerator. All the electrical measurements were performed at a base temperature ≈16 mK using standard ac lock-in techniques. How to cite this article: Cho, S. et al. Aharonov–Bohm oscillations in a quasi-ballistic three-dimensional topological insulator nanowire. Nat. Commun. 6:7634 doi: 10.1038/ncomms8634 (2015).